Determining the polarization state of an extreme ultraviolet free-electron laser beam using atomic circular dichroism Ultrafast extreme ultraviolet and X-ray free-electron lasers are set to revolutionize many domains such as bio-photonics and materials science, in a manner similar to optical lasers over the past two decades. Although their number will grow steadily over the coming decade, their complete characterization remains an elusive goal. This represents a significant barrier to their wider adoption and hence to the full realization of their potential in modern photon sciences. Although a great deal of progress has been made on temporal characterization and wavefront measurements at ultrahigh extreme ultraviolet and X-ray intensities, only few, if any progress on accurately measuring other key parameters such as the state of polarization has emerged. Here we show that by combining ultra-short extreme ultraviolet free electron laser pulses from FERMI with near-infrared laser pulses, we can accurately measure the polarization state of a free electron laser beam in an elegant, non-invasive and straightforward manner using circular dichroism. The advent of short-wavelength free-electron lasers (FELs) has enabled unique investigations of photo-induced processes. Non-linear phenomena and femtosecond time-resolved spectroscopy can be explored using high intensity extreme ultraviolet (XUV) and X-ray beams [1] , [2] , [3] . In addition, the ultra-short pulse duration and the high degree of spatial coherence of the X-ray FELs have enabled imaging experiments [4] , [5] , [6] aiming to determine the structure of a single biomolecule. Nearly all experiments to date have been carried out with linearly polarized short-wavelength FELs thereby precluding studies at high intensities and on systems where the result might depend on the target sensitivity to the helicity of the electric field. We are aware of only one FEL experiment with circularly polarized light [7] studying ferromagnetic, nanoscale spin order by imaging techniques. In this seminal work, linearly polarized light from the Linac Coherent Light Source was used together with a monochromator and transmission polarizer to obtain 58% circular polarization, albeit at the expense of a strong reduction in intensity. However, the FEL FERMI designed specifically to produce circularly polarized XUV radiation became available recently [8] , [9] . The use of these ultra-short circularly polarized XUV pulses is expected to lead to a series of breakthroughs in a number of associated domains, for example, spin-resolved features in atoms and molecules, symmetry-dependent characteristics of chiral biomolecules, the dynamics of magnetic properties of solids and the understanding of the secondary structure of proteins. Moreover, the extremely high intensity of the FEL source opens up a completely unexplored class of dichroism phenomena involving multi-photon processes at ultra-short wavelengths. Circular dichroism (CD) in photoemission is defined as the difference of the photoelectron yield for left and right circularly polarized ionizing radiation. For a non-zero CD to exist, it is necessary that the target has intrinsic or induced chiral properties, that is, physical properties that are not symmetric with respect to mirror reflection in one of the symmetry planes. Accordingly, CD in photoemission from solids has been widely used for the investigation of local magnetization and other properties of solids and surfaces (for example, refs 10 , 11 ). In atomic and molecular physics, circularly polarized photon beams have been applied for example in studies of electron spin-related phenomena and its polarization control [12] , [13] as well as of symmetry breaking in chiral molecules [14] , [15] . With FERMI many experimental techniques, already well established for applications of CD using synchrotron radiation, high order harmonics or optical lasers [16] , [17] , [18] , [19] , [20] , [21] , can now be extended to studies at FEL sources. Measurements which are currently limited by the signal to noise ratio or detection efficiency, have now become feasible and precise characterization of all FEL beam parameters will be crucial to making this powerful new source relevant, advantageous, effective and accessible to a wider scientific community. In this letter we report the experimental observation of CD in two-colour above threshold ionization of He atoms. The angle-resolved photoelectron spectra provide direct confirmation of the circular polarization of the FEL pulses and further enable the characterization of their polarization properties. Generally, CD in strong field single-colour multi-photon absorption by unpolarized target atoms or molecules is strictly zero [22] . However, in two-colour multi-photon ionization experiments CD is predicted to exist both in differential and integral electron yields [23] , [24] , [25] , [26] . Here we confirm this prediction while also demonstrating that this technique allows us to determine the degree of circular polarization of an intense XUV beam with high accuracy. Two-colour photoionization In the experiment, He atoms are ionized by XUV FEL radiation in the presence of an intense-near infra red (NIR) laser field. In the resulting photoelectron spectrum a series of lines, so-called sidebands, are observed on both sides of the normal photoline [27] , [28] . Since the sidebands are very sensitive to the spatial and temporal overlap and to the physical characteristics of both the XUV and NIR pulses, this type of experiment is widely used for studying multi-photon ionization dynamics [29] as well as for characterizing linearly polarized ionizing FEL pulses [30] . In the present study it is applied to the characterization of the polarization properties of the FEL beam. The CD is expected to be different in amplitude and sign for the central photoline and the sidebands [24] , [25] , [26] . The value of CD is directly proportional to the degree of circular polarization of the FEL beam and strongly depends on the intensity of the NIR field. The experimental results were obtained at the Low Density Matter (LDM) end-station of FERMI. Circularly polarized FEL pulses (48.4 eV, 100 fs, 80 μJ) were spatially and temporally overlapped with intense NIR pulses (784 nm, 175 fs, 30 μJ) in the interaction volume of a velocity map imaging (VMI) spectrometer ( Fig. 1 ). The NIR beam is produced by optically splitting the seeding laser beam and is introduced into the experimental chamber quasi-collinear with the XUV beam. For the measurement of the CD, the circular polarization of the ionizing XUV radiation was kept fixed (left-handed circular) and the polarization of the NIR-dressing field was switched from left- to right-handed by means of a rotating half wave plate—quarter wave plate combination. 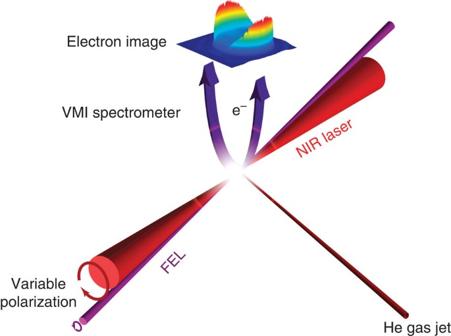Figure 1: Experimental setup used at the low density matter (LDM) end-station of FERMI. The free-electron laser beam is circularly polarized and is used with a fixed helicity. The infrared laser beam provides circular polarization of left- and right-handed helicity. Helium is injected into the merged beam section via a gas jet system. A velocity map imaging (VMI) spectrometer is used to determine the energy, intensity and angular distribution of the emitted-electron signal. Figure 1: Experimental setup used at the low density matter (LDM) end-station of FERMI. The free-electron laser beam is circularly polarized and is used with a fixed helicity. The infrared laser beam provides circular polarization of left- and right-handed helicity. Helium is injected into the merged beam section via a gas jet system. A velocity map imaging (VMI) spectrometer is used to determine the energy, intensity and angular distribution of the emitted-electron signal. Full size image Angle-resolved electron spectra and circular dichroism Typical angle-resolved electron spectra derived from the VMI image (see Fig. 1 ) are shown in Fig. 2a . The following points stand out in this photoelectron spectrum. About 11% of the total intensity is transferred from the main He 1 s photoline at 23.8 eV kinetic energy into the sidebands, which are separated by 1.58 eV from the main line. In agreement with the theoretical results ( Fig. 2b ), maximal electron emission is observed at 90°, that is, perpendicular to the beam propagation axis. The angular distribution of these two sidebands, which are caused by a two-photon process, is much narrower than that of the 1 s photoline, which predominantly arises from a one-photon process. 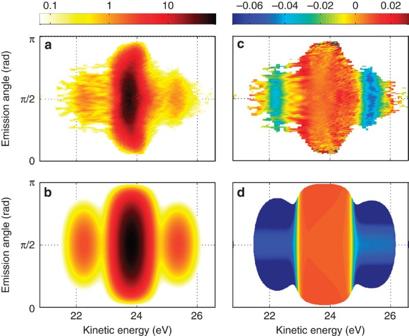Figure 2: Angle- and energy-resolved electron spectra and circular dichroism. Double differential cross section (a,b) and differential circular dichroism (c,d) in He 1 s photoionization at low-NIR laser intensity (7.3 × 1011W cm−2). Experimental results are shown in the upper panels, the results of simulations in the lower panels. The respective intensities are indicated by the colour scale on top of the graphs. Figure 2: Angle- and energy-resolved electron spectra and circular dichroism. Double differential cross section ( a , b ) and differential circular dichroism ( c , d ) in He 1 s photoionization at low-NIR laser intensity (7.3 × 10 11 W cm −2 ). Experimental results are shown in the upper panels, the results of simulations in the lower panels. The respective intensities are indicated by the colour scale on top of the graphs. Full size image The resulting CD is depicted in Fig. 2c and d for experiment and theory, respectively. Both reveal a clear dichroism of opposite sign for the main line and the sidebands. The observation of the CD demonstrates unequivocally that chirality is introduced into the (initially unpolarized atomic) system by the circularly polarized ionizing XUV radiation. The overlap with an NIR-dressing field of the same or the opposite helicity causes different probabilities for the transfer of electrons from the main line to the sidebands, that is, for the free-free transitions. Detailed consideration of the spectra provides more quantitative information ( Fig. 3 ). 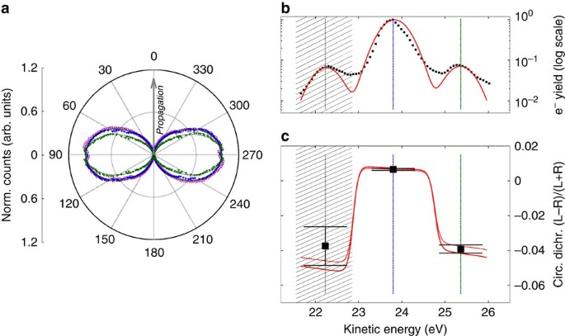Figure 3: Angular distribution and circular dichroism. (a) Polar representation of the angular distributions (normalized to the maximum) for the one-photon ionization of He (purple) and for the two-colour two-photon ionization leading to the main photoline (blue) and the sideband (green). Dashed-black curves are the best fitting of the experimental data with equation (1) and equation (2), respectively. (b) Experimental (black squares) and theoretical (solid red line) electron spectra. Dashed-vertical lines identify the position of the photoemission lines with the same colour code as in (a). (c) Comparison of the circular dichroism in the photoelectron emission derived from the experimental (black squares) and the theoretical (red lines) spectra at emission angles of (90±4)°; the red-dashed line represents a circular polarization of 90%. The squares represent the average value and the respective statistical error from the energy region corresponding to each photoemission line. The shaded area around the low-energy sideband was not taken into account for the analysis, since the overlap of this sideband with the main photoemission line in the VMI spectrum results in a large error bar (see text). Figure 3: Angular distribution and circular dichroism. ( a ) Polar representation of the angular distributions (normalized to the maximum) for the one-photon ionization of He (purple) and for the two-colour two-photon ionization leading to the main photoline (blue) and the sideband (green). Dashed-black curves are the best fitting of the experimental data with equation (1) and equation (2), respectively. ( b ) Experimental (black squares) and theoretical (solid red line) electron spectra. Dashed-vertical lines identify the position of the photoemission lines with the same colour code as in ( a ). ( c ) Comparison of the circular dichroism in the photoelectron emission derived from the experimental (black squares) and the theoretical (red lines) spectra at emission angles of (90±4)°; the red-dashed line represents a circular polarization of 90%. The squares represent the average value and the respective statistical error from the energy region corresponding to each photoemission line. The shaded area around the low-energy sideband was not taken into account for the analysis, since the overlap of this sideband with the main photoemission line in the VMI spectrum results in a large error bar (see text). Full size image The angular distribution of the He 1 s emission by circularly polarized FEL pulses in the absence of the NIR field is described by an asymmetry parameter β=+1.96±0.02 ( Fig. 3a ), which is almost identical to the theoretical value of β=+2 ( z -axis along the photon beam propagation direction) for this one-photon ionization process. In contrast, the angular distribution of the two-photon process (that is, the first high-energy sideband) is described by two asymmetry parameters, β 2 and β 4 (see Methods). The experimental values β 2 =+2.68±0.05 and β 4 =−0.71±0.04 are in excellent agreement with the simulation giving the theoretical values of +2.71±0.02 and −0.68±0.02, respectively. The degree of circular polarization is obtained by comparing the CD determined from the experimental- and the simulated-theoretical electron spectra ( Fig. 3b and c ) at emission angles of (90±4)°, where theory predicts maximal CD [25] . The measured amplitude of the CD averaged over the kinetic energy range of the high-energy sideband (25.2–26.1 eV) is −0.04±0.004. The CD of the low-energy sideband, though carrying the same information, is affected by the overlap with the signal from the main photoline in the two dimensional VMI image leading to a higher statistical error. Theory predicts a slightly larger negative CD for this sideband consistent with experiment. As follows from the analytical expressions in ref. 26 , this difference is caused by the fact that at low-NIR intensities the CD is inversely proportional to the kinetic energy of the electron. However, owing to the higher accuracy of the data only the high-energy sideband is considered in the further analysis. The experimental value for the CD is in excellent agreement with theory and is consistent with a degree of circular polarization P circ =0.95±0.05 for the XUV radiation reaching the interaction region. Any linear (or unpolarized) component in either NIR or XUV laser polarization would lead to a decrease in the value of the measured dichroism. Since the NIR beam is in a state of almost pure circular polarization (>99%), the magnitude of the circular polarization of the XUV beam can be determined with an error <5%. FERMI is predicted to produce 100% circular polarization, which reduces to 92% after transmission through the optics, in excellent agreement with the measurement. The method is therefore an important metrological tool for the determination of the degree of circular polarization, which is otherwise difficult to measure at the high power levels used here. Precise knowledge of the degree of polarization is indispensable for the quantitative analysis of dichroic phenomena and the detailed comparison with theoretical models. In the photoemission experiment, only the combined measurement of the angular distribution described by the asymmetry parameters β n and of the circular dichroism CD allows the unambiguous characterization of the polarization state of the XUV beam. Moreover, the sign of the dichroism is directly related to the relative helicity of both the NIR and XUV fields. The measured negative value for the dichroism indicates that the FEL beam was in a state of left-handed circular polarization (as defined from the point of view of the source), as expected from the settings of the undulator. The CD of the main line and its positive value is simply caused by polarization-dependent transfer of electrons to the sidebands. The small absolute value is affected by the imperfect overlap of the two pulses leading also to emission from the non-negligible fraction of undressed He atoms, which is taken into account in the simulation of the theoretical curve. In conclusion, we have shown that two-colour photoionization of an atom is a powerful and straightforward tool to determine the sign of the helicity and the magnitude of circular polarization of any XUV or indeed X-ray FEL beam with high accuracy. Moreover, the results confirm the theoretical prediction of CD in the two-colour multi-photon ionization of atoms, thereby paving the way towards a new research field in FEL-based science related to dynamical studies of dichroic effects. Experiment Angle-resolved two-colour multi-photon electron emission from atomic helium was measured at the LDM end-station of the seeded XUV FEL FERMI [31] using VMI spectrometry. Circularly polarized XUV pulses of hv =48.4 eV (25.6 nm), with a bandwidth of about 94 meV (0.05 nm) and a duration of about 100 fs were delivered by Advanced Planar Polarized Light Emitter (APPLE II) -type undulators via the Photon Analysis Delivery and REduction System (PADRES) [32] . The XUV pulse duration T FEL was deduced from its dependence on the harmonic number n h in a seeded FEL, which is given by T FEL = T seed × ( n h ) −1/3 (ref. 33 ), and using for present experiment the measured seed pulse duration T seed =210 fs and the 10th harmonics. The average pulse energy was 80±10 μJ with a repetition rate of 10 Hz. Active mirrors in Kirkpatrick–Baez configuration focused the FEL pulses to a spot size of about 50 μm diameter (Full width at half maximum). Taking into account the theoretical overall transmission of all optical components in the beamline (about 60%), average intensities up to 10 13 W cm −2 were reached in the interaction region. Circularly polarized NIR pulses from a Ti:Sa laser (784 nm; 1.58 eV), with a bandwidth of 13 nm (Full width at half maximum), a duration of 175 fs and pulse energies of 30 μJ were used in the experiment. With a spot size of 150±20 μm diameter a maximal intensity of (7.3±1.6) × 10 11 W cm −2 could be achieved. A higher NIR pulse energy (750 μJ) was used for the initial optimization of the two-colour signal. However, the lower intensity was applied for the experiment, since at this intensity only the first sideband was observed in the electron spectra enabling the straightforward interpretation of the CD in the two-colour ionization. The pulse energy was adjusted by a polarizer-based variable attenuator. Since the laser pulses are derived by splitting the FEL-seeding pulses, they provide almost jitter-free operation and very good two-colour synchronization. The FEL and the NIR pulses were overlapped in time and space in the centre of the experimental chamber. The spatial overlap was determined by visual inspection of the images of both beams on an Yttrium Aluminium Garnet monitor insertable into the interaction region. The temporal overlap was controlled by a delay stage in the NIR-laser delivery system and was optimized using first a coaxial cable antenna and then directly the two-colour two-photon signals. The VMI spectrometer includes a 75 mm diameter imaging quality multi-channel plate (MCP) stack with a high quality camera for the MCP image readout [31] . Its electron optics were set to work optimally for the kinetic energies of the He 1s electrons given by E kin = E hν (48.4 eV)− E He(1 s) (24.6 eV)=23.8 eV. Calibration was achieved by analyzing the electron emission of different noble gas targets at various photon energies. A pulsed, supersonic helium injection beam produced with a commercial Even–Lavie valve (aperture 100 μm) was used to provide sufficient gas density (about 10 12 atoms per cm 3 ) in the interaction region for a shot-to-shot analysis of the VMI-spectra [31] . Data analysis The sCMOS camera readout acquires pictures of two dimensional projections of electron angular distributions with a 2,560 × 2,160 pixels (6.5 μm) resolution [31] . These images (see for example, Fig. 1 ) are transformed into three-dimensional momentum distributions with full angular reconstruction of the electron emission by applying an Abel transformation [34] . The CD was derived by subtraction of the three-dimensional images of differently handed circular polarizations normalized by the sum of both contributions. The helium 1 s electron line as well as the sidebands were analyzed for their angular distributions. Since the FEL as well as the NIR laser were circularly polarized during the experiments, the propagation axis of the light is the symmetry axis for the electron angular distribution. The angular distribution of the photoelectrons emitted by a one-photon process is described by for the corresponding two-colour two-photon process by where the angle θ is measured with respect to the propagation axis of the ionizing FEL beam. P n (cos θ ) denotes the Legendre polynominal of n th order and β, β 2 and β 4 are the asymmetry parameters. Modelling For simulations we use the theoretical model developed in papers [25] , [26] , which is based on the Strong Field Approximation (SFA) [35] . We consider the process within the first-order time-dependent perturbation theory and use the rotating wave approximation for the XUV photon—electron interaction. Then the photoionization amplitude can be presented as (atomic units are used throughout unless otherwise indicated) where is the envelope of the XUV pulse, w X is its mean frequency, E b is the binding energy (positive) of the electron, Ψ 0 and Ψ f are the initial atomic and final ionic wave functions, respectively, and is the dipole operator for right (+) and left (−) circularly polarized XUV radiation. The wave function in equation (3) describes the ‘dressed’ photoelectron in the laser field, which is characterized by the final (asymptotic) momentum . Within the SFA, the wave function of the photoelectron is represented by the non-relativistic Volkov wave function [36] : Here is the Volkov phase with being the vector potential of the NIR-laser field, different for right and left circularly polarized light. (For more details see ref. 26 .) The square of the amplitude equation (3) determines the differential cross section. The CD in the angular distribution is usually characterized by the relative value: where superscript LL marks the amplitude when both XUV and NIR pulses are left circularly polarized, while superscript LR indicates that the NIR field is right circularly polarized. The theoretical differential cross sections and in equation (6) are calculated for spatially homogeneous pulses with realistic temporal shapes. To compare the theoretical and the experimental results the presence of low intensity wings in the FEL beam not overlapping with the IR beam as well as the IR field inhomogeneity had to be taken into account. The latter is owing to the spatial distribution of the IR intensity in the FEL beam and to the imperfect overlap of the two beams. For simulating these experimental conditions, we have calculated the double differential cross section for various IR peak intensities. The modelled cross sections are then calculated from the superposition of contributions coming from areas with different IR intensities. The uncertainty in the overlapping geometry is accounted for and propagated into the experimental and theoretical error bars for the asymmetry parameters and the CD. How to cite this article: Mazza, T. et al. Determining the polarization state of an extreme ultraviolet free-electron laser beam using atomic circular dichroism. Nat. Commun. 5:3648 doi: 10.1038/ncomms4648 (2014).